Crystal structure and its bearing towards an understanding of key biological functions of EpCAM EpCAM (epithelial cell adhesion molecule), a stem and carcinoma cell marker, is a cell surface protein involved in homotypic cell–cell adhesion via intercellular oligomerization and proliferative signalling via proteolytic cleavage. Despite its use as a diagnostic marker and being a drug target, structural details of this conserved vertebrate-exclusive protein remain unknown. Here we present the crystal structure of a heart-shaped dimer of the extracellular part of human EpCAM. The structure represents a cis -dimer that would form at cell surfaces and may provide the necessary structural foundation for the proposed EpCAM intercellular trans -tetramerization mediated by a membrane-distal region. By combining biochemical, biological and structural data on EpCAM, we show how proteolytic processing at various sites could influence structural integrity, oligomeric state and associated functionality of the molecule. We also describe the epitopes of this therapeutically important protein and explain the antigenicity of its regions. Cell surface molecules, including cell adhesion molecules, are critically involved in sensing the surroundings of cells. A member of this diverse group of proteins is the epithelial cell adhesion molecule (EpCAM, CD326), a type I transmembrane (TM) glycoprotein of the small GA733 protein family named after the monoclonal antibody raised to the human gastric adenocarcinoma line [1] . In contrast to low expression in normal simple epithelia, EpCAM is frequently expressed at high levels in various epithelial cancers (carcinomas) [2] and in undifferentiated human embryonic stem cells [3] , [4] . Elevated EpCAM levels in carcinomas are exploited by several anti-tumor approaches, which deploy EpCAM for drug targeting (reviewed in ref. 5 ) and a trifunctional bispecific anti-EpCAM anti-CD3 antibody is already approved for use in EU (Catumaxomab) [6] . Several mutations within the EPCAM gene result in truncated or misfolded protein, which is accompanied by incorrect cellular EpCAM localization; these mutations are directly associated with congenital tufting enteropathy (CTE), a rare and severe form of diarrhoea (reviewed in ref. 7 ). Initially, EpCAM was postulated to be involved in calcium-independent cell–cell adhesive contacts, which do not resemble the classical junction contacts [8] , [9] , [10] . It was demonstrated that the weak homotypic adhesive function is associated with formation of oligomeric adhesion units in the intercellular space via direct cis - and trans -interactions of the larger extracellular parts (EpEX, 27 kDa) [11] , [12] . These units are believed to be anchored to the actin cytoskeleton via interaction of the intracellular tail (EpIC, 3 kDa) with α-actinin [13] . However, it was also demonstrated that EpCAM can have a negative effect on the strength of cell–cell adhesion mediated by E-cadherin thereby promoting cell migration and motility [14] , [15] . EpCAM also plays an important role in the formation of functional tight junctions and regulation of epithelial integrity via direct interaction with claudin-7 (refs 16 , 17 , 18 ). Recently, it was discovered that EpCAM functions as a signalling molecule [19] . Here, the formation in intercellular EpCAM oligomers appears to be a prerequisite for triggering a proliferation-enhancing signalling cascade starting with regulated intramembrane proteolytic cleavage of EpCAM by a membrane protease complex releasing the EpEX and EpIC. The complex of EpIC, FHL2 and β-catenin is then translocated to the nucleus where it associates with LEF1 and directly affects cell proliferation at transcriptional level [19] , [20] . However, the outlined aspects of EpCAM biology are far from being well-defined, especially from the structural point of view, since to date no representative structure was available to interpret the experimental observations. Here, we present the structure of a non-glycosylated mutant form of EpEX (EpEXΔ) at 1.86-Å resolution, a first and exemplary structure of the unique GA733 protein family. In this structure, EpEXΔ forms a cis -dimer corresponding to a half of the proposed trans -tetrameric intercellular unit. We reveal the cis -dimerization interface between the two subunits involving the thyroglobulin type-1A (TY) domain and thereby describe a novel role of the versatile TY protein module. EpCAM cis -dimer could be additionally stabilized by interaction of the TM helices of the two cis -oriented subunits as we explore by molecular dynamics (MD) simulations. We show that the lateral protein surfaces of the wt EpCAM cis -dimer are partially covered with glycan chains as inferred from the position of known N -glycosylation sites. The structure explains the high antigenicity of the surface-exposed small amino-terminal domain that harbours conformational epitopes of the majority of anti-EpCAM antibodies. We provide a model of the trans -tetrameric intercellular unit where the trans -interactions involve the glycan-free membrane-distal platform-like surface of EpEXΔ. Finally, we comment on the design of efficient EpCAM-targeted binder molecules and explain the detrimental effect of CTE-causing mutations on EpCAM structure and function. Structure determination We determined the crystal structure of the human mutant EpEXΔ in which three Asn-to-Gln mutations were introduced to abolish N -linked glycosylation of Asn74, Asn111 and Asn198 residues ( Fig. 1a ). These mutations enabled us to obtain a highly homogenous protein sample ( Supplementary Fig. 1a ). After extensive diffraction screening, a complete and highly redundant data set was recorded from a single crystal at 1.54 Å wavelength ( Supplementary Fig. 1b ). The data were indexed in the C 2 space group with unit-cell lengths of 88.0 × 50.4 × 67.8 Å. 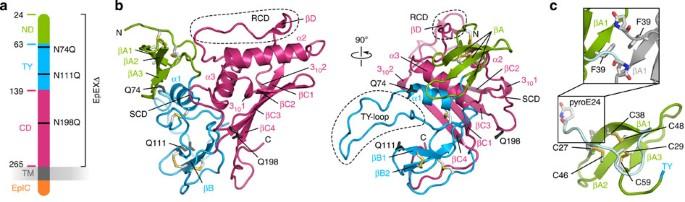Figure 1: EpEXΔ subunit structure. (a) EpEXΔ is composed of N-domain (ND, green), TY domain (blue) and CD (dark pink). It lacks the TM and intracellular part (EpIC) of full-length EpCAM. In addition, it contains threeN-glycosylation-abolishing mutations (indicated by black lines). (b) Cartoon representation of the complete EpEXΔ chain contained in the asymmetric unit shown in two different orientations. Color coding is the same as ina. Secondary structure elements are labelled as they appear along the polypeptide chain from N to C terminus (for example, βA for β-sheet A, βA1 for first strand in βA sheet, α1 and 3101 for first α- and 310-helix, respectively). The three glutamine residues (N-glycosylation abolishing mutations) are shown as black sticks. (c) ND shown as cartoon. N-terminal pyroGlu residue (pyroGlu24), Phe39, and all disulphide bridges are shown as sticks. The N-terminal region tethered to the βA sheet is coloured in pale cyan. Zoomed-in part shows contact between ND (green) and its copy from the adjacent asymmetric unit (grey). Initial phases were calculated using the anomalous signal of intrinsic sulphur atoms, and the structure was solved and refined at 1.86 Å-resolution ( Table 1 ). The overall quality of the electron density map was high except for some surface regions, which display a higher B-factor ( Supplementary Fig. 1c ). An extended blob of electron density that could not be assigned to the EpEXΔ polypeptide chain was modelled as a crystallization additive n-decyl-β- D -maltopyranoside, bound in a narrow hydrophobic pocket ( Supplementary Fig. 2 ). Figure 1: EpEXΔ subunit structure. ( a ) EpEXΔ is composed of N-domain (ND, green), TY domain (blue) and CD (dark pink). It lacks the TM and intracellular part (EpIC) of full-length EpCAM. In addition, it contains three N -glycosylation-abolishing mutations (indicated by black lines). ( b ) Cartoon representation of the complete EpEXΔ chain contained in the asymmetric unit shown in two different orientations. Color coding is the same as in a . Secondary structure elements are labelled as they appear along the polypeptide chain from N to C terminus (for example, βA for β-sheet A, βA1 for first strand in βA sheet, α1 and 3 10 1 for first α- and 3 10 -helix, respectively). The three glutamine residues ( N -glycosylation abolishing mutations) are shown as black sticks. ( c ) ND shown as cartoon. N-terminal pyroGlu residue (pyroGlu24), Phe39, and all disulphide bridges are shown as sticks. The N-terminal region tethered to the βA sheet is coloured in pale cyan. Zoomed-in part shows contact between ND (green) and its copy from the adjacent asymmetric unit (grey). Full size image Table 1 Data collection and refinement statistics. Full size table Overall subunit structure of human EpEXΔ The polypeptide chain of EpEXΔ is folded into three domains (ND, TY and CD, see Fig. 1a ) arranged in a triangular fashion where each domain contacts the other two ( Fig. 1b ). The first residue immediately after the signal peptide cleavage site (Gln24) is modified to pyroglutamate (pyroGlu), which is a common modification of an extracellular N-terminal and has already been observed in recombinant EpEX [21] ( Fig. 1c ). The small and compact disulphide-rich N-terminal domain of 39 amino-acid residues (N-domain or ND, pyroGlu24-Leu62; green in Fig. 1 ) lacks an extensive hydrophobic core. Instead, its structure is stabilized by three closely spaced disulphide bridges (Cys27-Cys46, Cys29-Cys59 and Cys38-Cys48), which tether the N-terminal region of the chain (pyroGlu24-Leu34) to the concave face of a curved three-stranded β sheet with strand order 1-2-3 (βA, Fig. 1c ). The disulphide bond pattern observed in our structure confirms the previously determined cysteine bonding [21] . A similar triple disulphide bond pattern is found in other small protein domains, for example in the Cripto CFC domain [22] . According to the alignment of 3D structures in the PDB database [23] , the ND domain is most similar to the WW protein module [24] . However, there are considerable differences: (i) ND lacks the two highly conserved tryptophan residues found in WW modules, and (ii) WW modules do not contain disulphide bridges and lack the N-terminal region present in ND. The solvent-exposed regions of the ND are negatively charged (N-terminal region) or polar (convex side of the βA sheet) with an exception of Phe39 within the FVNNN sequence motif (conserved in primates; Supplementary Fig. 3a ). In our crystal structure, the side chains of two Phe39 residues from adjacent asymmetric units are involved in parallel-displaced π–π interactions (inset in Fig. 1c ). ND is followed by the TY domain (Ala63-Arg138; blue in Fig. 1 ), which is a TY module with a characteristic fold stabilized by an evolutionarily conserved disulphide bridge pattern (Cys66-Cys99, Cys110-Cys116 and Cys118-Cys135 as numbered in EpCAM) [21] and a CWCV sequence motif within the βB ribbon [25] . The secondary structure elements (α1 helix and βB ribbon) and neighbouring regions of the polypeptide chain form a small hydrophobic core additionally stabilized by the three disulphide bridges. The region between the α1 helix and the βB ribbon of the TY domain protrudes as a loop (TY loop) from the otherwise compact EpEXΔ molecule ( Fig. 1b ). The third domain (carboxy-terminal domain, C-domain or CD, Val139-Lys265; dark pink in Fig. 1 ) belongs to the α+β fold class. The helices are clustered on one side of the slightly twisted βC sheet, which forms a negatively charged polar concave surface on the side of the EpEXΔ molecule ( Fig. 1b ). Here, the two amphipathic α helices are on the hydrophobic convex side within the regions connecting the β strands of the βC sheet. This fold resembles the fold of some unrelated protein domains, for example, the RNA binding domain of Bacillus subtilis YxiN [26] and the mature ectodomain of human receptor-type protein tyrosine phosphatase IA-2 (ref. 27 ). The major differences are in the loop regions connecting the secondary structure elements where in EpEXΔ the most prominent part is the region connecting the α3 helix with the βC sheet (Lys221-Thr247). The central part of this region (His227-Gln239, ‘ridge on CD’ or RCD) contains a stretch of polypeptide chain that runs in parallel to the α2 helix and a short β hairpin. In addition, two residue triplets (Pro178-Phe180 and Pro244-Gln246) within CD have a 3 10 conformation resulting in two interlocked tight turns on each side of the βC sheet (3 10 1 and 3 10 2 in Fig. 1b ). Region Lys202-Asn205 (‘side loop on CD’ or SCD) does not have a well-defined electron density indicating some flexibility in this surface-exposed turn ( Supplementary Fig. 1c ). The EpEX cis -dimer In vivo , EpCAM forms a cis -dimer where the two subunits laterally interact on the cell surface [11] , [12] . Indeed, EpEXΔ crystallized as a dimer, which is formed by two EpEXΔ chains from adjacent asymmetric units related by the crystallographic twofold symmetry axis ( Fig. 2a,c ). The dimeric form is also present in solution as demonstrated by crosslinking ( Fig. 3a ) and size-exclusion chromatography [28] . The extensive buried surface area of 1,980 Å 2 (per subunit) with a solvation free energy gain on formation of the interface of −8.6 kcal mol −1 and a P value of 0.358 as calculated by PISA [29] indicates strong and specific interaction. The interaction surface represents 14% of the subunit surface area; the upward-oriented C-terminal region Met261-His266 was excluded from this calculation (see below). The most prominent interaction region is formed by the TY loop of one subunit and a concave βC sheet of the other subunit (yellow in Fig. 2c ). Specifically, Arg80, Arg81 and Lys83 of the TY loop of one subunit are involved in electrostatic interactions with the acidic patch formed by Glu147, Glu187 and Asp194 of the βC sheet of the other subunit ( Fig. 2b ). The side chain of Gln74, which in wt EpCAM corresponds to glycosylated Asn74, is oriented towards the solvent and is not involved in the dimerization interactions. 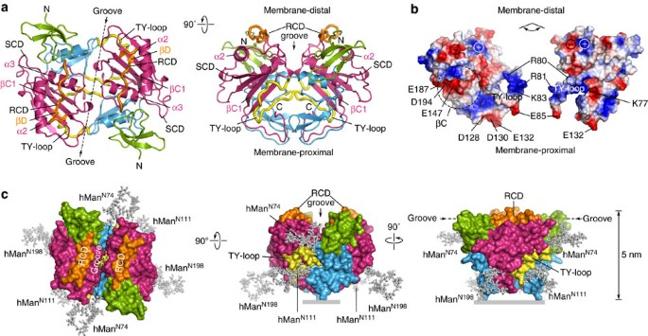Figure 2: Structure of EpEXΔcis-dimer. (a) Cartoon representation of EpEXΔcis-dimer in two different orientations (top, side). (b) The molecular surface of EpEXΔcis-dimer, color coded by electrostatic potential. Subunits are moved apart and rotated to reveal the oppositely charged interaction regions. (c) Molecular surface of EpEXΔcis-dimer with modelled high-mannose chains atN-glycosylation sites ofwtEpCAM (Asn74, Asn111 and Asn198) shown in three different orientations relatively to the membrane (grey bar). The three domains of each subunit ina,care color coded as inFig. 1. Ina,c, the first long loop of TY domain (TY loop) and the RCD within C-domain are shown in yellow and orange, respectively. For clarity, the C-terminal region of EpEXΔ (from Met261 to Lys265 plus His266) is not shown inb,c. Figure 2: Structure of EpEXΔ cis -dimer. ( a ) Cartoon representation of EpEXΔ cis -dimer in two different orientations (top, side). ( b ) The molecular surface of EpEXΔ cis -dimer, color coded by electrostatic potential. Subunits are moved apart and rotated to reveal the oppositely charged interaction regions. ( c ) Molecular surface of EpEXΔ cis -dimer with modelled high-mannose chains at N -glycosylation sites of wt EpCAM (Asn74, Asn111 and Asn198) shown in three different orientations relatively to the membrane (grey bar). The three domains of each subunit in a , c are color coded as in Fig. 1 . In a , c , the first long loop of TY domain (TY loop) and the RCD within C-domain are shown in yellow and orange, respectively. For clarity, the C-terminal region of EpEXΔ (from Met261 to Lys265 plus His266) is not shown in b , c . 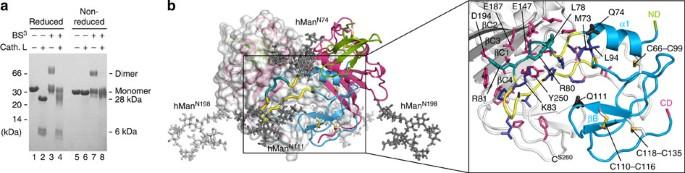Figure 3: Role of TY loop incis-dimerization. (a) SDS–PAGE analysis of crosslinked intact and cathepsin L-cleaved EpEXΔ samples under reducing and non-reducing conditions. Cleavage with cathepsin L results in 6 and 28 kDa fragments connected by a disulphide bond. Only intact EpEXΔ forms a stable dimer, which can be crosslinked by BS3. (b) Overall view (bottom) of the model of glycosylated EpEXcis-dimer shows that the access to the protease-sensitive Leu78-Gly79-Arg80-Arg81 (dark teal ribbon) within the TY domain between is partially obscured by glycan residues (grey sticks). TY loop and ND, TY and CD domains are color coded as inFig. 2. Detailed view (top) of TY-loop residues (dark purple) interacting with residues of βC sheet (grey, side chains within 4 Å of TY loop shown in dark pink). The Arg80 and Arg81 (dark teal sticks) interact with Asp194, Glu154 and Glu147. Gln74 and Gln111 (black sticks) introduced by glycosylation-abolishing mutations within TY correspond to glycosylated Asn residues inwtEpEX. The three disulphide bonds of TY are shown as sticks. Under non-reducing conditions, the 6 and 28 kDa fragments (ND plus α1 and the rest of TY plus CD, respectively) remain connected by the Cys66-Cys99 bond. For clarity, the C-terminal region of EpEXΔ (from Met261 to Lys265 plus His266) is not shown. Full size image Figure 3: Role of TY loop in cis -dimerization. ( a ) SDS–PAGE analysis of crosslinked intact and cathepsin L-cleaved EpEXΔ samples under reducing and non-reducing conditions. Cleavage with cathepsin L results in 6 and 28 kDa fragments connected by a disulphide bond. Only intact EpEXΔ forms a stable dimer, which can be crosslinked by BS 3 . ( b ) Overall view (bottom) of the model of glycosylated EpEX cis -dimer shows that the access to the protease-sensitive Leu78-Gly79-Arg80-Arg81 (dark teal ribbon) within the TY domain between is partially obscured by glycan residues (grey sticks). TY loop and ND, TY and CD domains are color coded as in Fig. 2 . Detailed view (top) of TY-loop residues (dark purple) interacting with residues of βC sheet (grey, side chains within 4 Å of TY loop shown in dark pink). The Arg80 and Arg81 (dark teal sticks) interact with Asp194, Glu154 and Glu147. Gln74 and Gln111 (black sticks) introduced by glycosylation-abolishing mutations within TY correspond to glycosylated Asn residues in wt EpEX. The three disulphide bonds of TY are shown as sticks. Under non-reducing conditions, the 6 and 28 kDa fragments (ND plus α1 and the rest of TY plus CD, respectively) remain connected by the Cys66-Cys99 bond. For clarity, the C-terminal region of EpEXΔ (from Met261 to Lys265 plus His266) is not shown. Full size image The plausible orientation of EpEXΔ (as a part of the full-length EpCAM) relative to the cell membrane can be inferred by the position of N and C termini. In full-length EpCAM, the C terminus of the extracellular part is connected to the TM region, suggesting that this is the membrane-proximal part. Since both C termini in the EpEXΔ structure are on the same side of the dimer (side orientation in Fig. 2a ), we conclude that this dimer architecture represents extracellular parts of two EpCAM molecules on the surface of the same cell, and will refer to it as a cis -dimer. The membrane-proximal part encompasses the TY domain and the βC sheet of the C-domain ( Fig. 2a ) and forms a tip of the cis -dimer with a net negative charge (Glu85, Asp128 and 130, Glu132; Fig. 2b ) suggesting that it is not in contact with the central hydrophobic part of the lipid bilayer as part of the full-length membrane-embedded EpCAM. However, the C-terminal part of the EpEXΔ chain (from Met261 to Lys265 plus the first histidine residue His266 of the His 6 -tag) is curved upwards ( Fig. 2a ) and forms several polar contacts with parts of TY domains from both subunits ( Supplementary Fig. 4 ). In wt glycosylated EpEX such conformation could be sterically hindered by the glycan chain attached to the Asn111 within the βB of TY ( Fig. 2c ). In full-length wt EpCAM, this region is probably oriented ‘downwards’ as discussed in the section regarding the TM helix (below). The membrane-distal part of this cis -dimer forms a central groove edged by the two RCDs and diagonally protruding small N-domains ( Fig. 2a,c ). The inner surface of the groove is formed by diametrically opposing basic and acidic patches (plus and minus sign labels in Fig. 2b ). The EpEXΔ cis -dimer has the shape of a heart (view along the RCD) or trapezoid (view perpendicularly to RCD) with a narrowed membrane-proximal part ( Fig. 2c ). Such dimer would protrude ~5 nm from the cell surface. In humans, EpCAM is glycosylated on the three N -glycosylation sites: Asn74 at the start of the TY loop, Asn111 within βB of the TY, and Asn198 between βC and α3 within CD [30] . The glycosylation is heterogeneous and at least one site is occupied by a high-mannose chain [31] . The EpEXΔ structure with modelled high-mannose chains attached at all three sites shows that the glycans partially cover the sides of the membrane-proximal part (Asn111 and Asn198) or are located at the start/end of the central groove of membrane-distal part of the cis -dimer (Asn74; Fig. 2c ). The top membrane-distal part of the molecule formed by RCD and ND is free of glycan chains. Cleavage within TY disrupts the cis -dimer In vivo , full-length glycosylated EpCAM (~38 kDa) is proteolytically processed within a protease-sensitive region containing the dibasic site Arg80-Arg81 of the TY loop [32] , [33] , [34] . The resulting 6 kDa N-terminal and 32 kDa C-terminal fragments remain connected by a disulphide bond. In EpEXΔ, the larger C-terminal fragment would correspond to a 28 kDa fragment lacking the TM and the cytosolic part. To resolve the impact of this cleavage on structural integrity of EpCAM, we generated the cleaved form of EpEXΔ and analysed its dimerization potential by chemical crosslinking. The cleaved form was generated by treating the purified EpEXΔ (~33 kDa, lanes 1 and 5 in Fig. 3a ) with human cathepsin L. The major cleavage site was at Gly79-Arg80 with a minor cleavage also at Leu78-Gly79, that is, both within the same protease-sensitive region as reported previously using several other proteases [34] . In the absence of crosslinker and under non-reducing conditions, the 6 and 28 kDa fragments remain connected via a disulphide bond (lane 6 in Fig. 3a ). However, under reducing conditions, the 6 kDa fragment is released from the rest of the molecule (28 kDa, lane 2 of Fig. 3a ). A band at the mass corresponding to a EpEXΔ dimer (~66 kDa) was observed only with crosslinked intact EpEXΔ (lanes 3 and 7 in Fig. 3a ). Although part of cleaved and crosslinked EpEXΔ has under reducing conditions (lane 4) similar electrophoretic mobility than non-cleaved EpEXΔ such molecule cannot form a dimer anymore (lanes 4 and 8 in Fig. 3a ). Cleavage using glycosylated EpEX as a substrate resulted in the same fragment pattern as for the EpEXΔ ( Supplementary Fig. 5 ). Also, the same fragment pattern could be generated using cathepsin K, which also cleaves at the Gly79-Arg80 site. In the structure of the EpEXΔ cis -dimer, the side chain of Leu78 is oriented towards the solvent while the basic side chains of Arg80 and Arg81 of one subunit are oriented towards the βC sheet of the CD of the other subunit where they are involved in cis -dimer-stabilizing interactions with acidic (Arg80 with Glu147, Arg81 with Asp194) and other residues (Val190, Gln246 and Leu248; Fig. 3b ). In the EpEX cis -dimer, access to the cleavage site Leu78-Gly79-Arg80 could be partially hindered by glycan chains attached to Asn74 (at the beginning of TY loop) and Asn111 (within turn in βB) as inferred from the model of glycosylated EpEX ( Fig. 3b ). Role of TM helix in cis -dimerization In the crystal structure of the EpEXΔ cis -dimer, the C termini are curved upwards ( Fig. 2a ). However, in full-length, membrane-anchored EpCAM, the C-terminal region of the extracellular part must be oriented towards the membrane to be connected to the TM part. Considering that the cell surface full-length EpCAM is a cis -dimer as inferred from the crystal structure and from the crosslinking experiments [12] , such downward orientation would bring the C-terminal regions of the two subunits into close proximity. Therefore, it is plausible to assume that also the TM part (single helix per chain) forms a dimer with potential to additionally stabilize the EpCAM cis -dimer. To investigate the dimerization propensity of the EpCAM TM helix, we performed coarse-grained (CG) MD simulations of two modelled EpCAM TM helices embedded in a lipid bilayer. The two EpCAM TM helices were allowed to diffuse freely within the bilayer patch from their initial positions separated by 50 Å. The plot of interhelical distance versus time in each of the simulations shows that once the two helices encountered each other the helix dimer stayed stable throughout the simulation (runs 1 and 3–6 in Fig. 4a ). In one of the simulation runs, the two helices did not encounter each other (run 2 in Fig. 4a ). In this run, the interhelical crossing angle distribution is flattened and centred near zero degrees as compared with two sharp peaks of bimodal interhelical crossing angle distribution observed in the other runs ( Fig. 4b ). Here, the two peaks of the crossing angle distribution are at −30° and +30°, corresponding to right- and left-handed packing. Higher frequencies of the −30° peak indicate that a right-handed packing is favored. Preference for certain crossing orientation has already been observed in CG MD simulations of the wt glycophorin A TM helix dimer; in contrast to this, the glycophorin A TM dimer disruptive mutants showed a more uniform distribution between the right- and left-handed crossing angle [35] . In a representative CG model of a right-handed EpCAM TM helix dimer, the two helices are arranged almost symmetrically and the crossing region encompasses the residues Val276-Val280 ( Fig. 4c ). Here, the Ile277 side chain of one helix locks into a pocket formed by side chains of Val276, Val279 and Val280 from the other helix. On the basis of these results, we predict that the EpCAM TM helix has a propensity to form a dimer when embedded in a lipid bilayer. 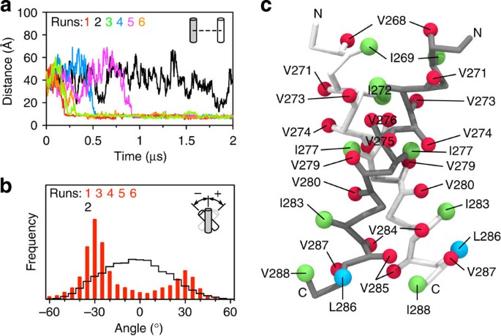Figure 4: TM helix dimerization contributes to stability of EpCAMcis-dimer. (a) Interhelical distance calculated from six CG MD simulations started from the same initial state. (b) Interhelical crossing angle distribution in combined simulation runs 1 and 3–6 (red), and run 2 (black). For combined runs only those parts where the two helices formed a dimer were used for calculation. (c) Representative CG dimer model TM helices of EpCAM calculated by MD simulation. Backbones of the two helices are shown as light and dark gray sticks. CG side chains of leucine, isoleucine and valine residues are shown as blue, green and red spheres, respectively. Labels follow residue numbering in full-length EpCAM. Figure 4: TM helix dimerization contributes to stability of EpCAM cis -dimer. ( a ) Interhelical distance calculated from six CG MD simulations started from the same initial state. ( b ) Interhelical crossing angle distribution in combined simulation runs 1 and 3–6 (red), and run 2 (black). For combined runs only those parts where the two helices formed a dimer were used for calculation. ( c ) Representative CG dimer model TM helices of EpCAM calculated by MD simulation. Backbones of the two helices are shown as light and dark gray sticks. CG side chains of leucine, isoleucine and valine residues are shown as blue, green and red spheres, respectively. Labels follow residue numbering in full-length EpCAM. Full size image Model of EpCAM intercellular unit It is believed that EpCAM-mediated adhesion and signalling involves formation of intercellular trans -oligomers. We used docking to generate a model of a trans -tetrameric intercellular unit based on our crystal structure of the cis -dimer together with available experimental data: (i) the ND is not required for intercellular adhesion [12] , (ii) juxtaposed cell membranes at EpCAM adhesion sites are separated by 10–14 nm [10] and (iii) lack of EpCAM N -glycosylation has no influence on its adhesive properties [12] . Our model ( Fig. 5 ) satisfies the outlined requirements, also in terms of intermembrane separation where the extended C-terminal region contributes an additional 1 nm separation to the 5 nm membrane-to-tip distance of the EpEXΔ cis -dimer ( Fig. 2c ). The trans -interaction surface is formed by the membrane-distal parts of the EpEXΔ dimer including the RCD while the glycan residues project sideways from the rhombohedral-shaped trans -tetramer ( Fig. 5 ). 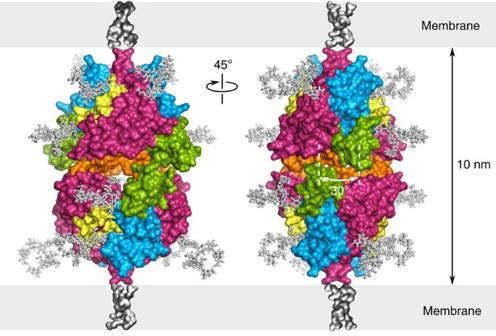Figure 5: Model of atrans-tetrameric intercellular unit. In the most probable relative orientation, the angle between the twocis-dimers is 30°. The model is shown in two different orientations with modelled high-mannose glycan chains (as inFig. 2c) and dimers of the TM parts (as inFig. 4b). The C termini were modelled in an extended conformation. EpEX domains and regions (TY loop and RCD) are color coded as inFig. 2. Figure 5: Model of a trans -tetrameric intercellular unit. In the most probable relative orientation, the angle between the two cis -dimers is 30°. The model is shown in two different orientations with modelled high-mannose glycan chains (as in Fig. 2c ) and dimers of the TM parts (as in Fig. 4b ). The C termini were modelled in an extended conformation. EpEX domains and regions (TY loop and RCD) are color coded as in Fig. 2 . Full size image The presented EpEXΔ structure reveals that the extracellular part of EpCAM is folded in a compact shape and is not extending from the cell surface in a linear way as portrayed in early models. In the crystal structure, EpEXΔ is present as a dimer and on the basis of a large interaction surface and orientation of the C termini, we postulate that this form represents a cis -dimeric cell surface form of EpCAM. The dimerization crucially depends on the TY domain, which adds dimerization to the functional repertoire of this versatile protein module besides cysteine protease inhibition as in p41 invariant chain [36] , inhibition and substrate behaviour as in testican-1 (ref. 37 ), and binding of insulin-like growth factor 1 as in IGF binding proteins [38] . The first loop of the TY module is the most divergent region of TY domains from various protein architectures and represents one of the functional determinants of these modules [39] . The TY domain of EpCAM does not inhibit cysteine cathepsins (M.P. and B.L., unpublished data); one of the more obvious reasons are the steric hindrances imposed by the long first loop that might prevent its binding to the active site cleft of the protease. Instead, this first loop (TY loop) is directly involved in interactions with the CD of the other subunit in the same dimer. This cis -dimer could be additionally stabilized by extension of the dimerization interface to the TM part with implications in intramembrane interactions of EpCAM with other proteins and vice versa . Moreover, the intramembrane dimerization potential of EpCAM TM parts could be influenced by the composition of the lipid bilayer. In our MD simulations, we used the simple 1-palmitoyl-2-oleoylphosphatidylcholine lipid bilayer; however, it has been reported that a complex of EpCAM and claudin-7 is recruited to the complex glycolipid-enriched tetraspanin microdomains [40] , which are known modifiers of adhesion and signalling functions of TM molecules. The key role of TY loop in dimerization interactions is also illustrated by the TY loop-cleaved form of EpEXΔ, which is not able to form a stable cis -dimer anymore. However, the cleavage site does not seem to be easily accessible to proteases since it is directly involved in cis -dimerization interactions. Even more, in glycosylated EpEX (model in Fig. 3b ) the access to the cleavage site could be sterically hindered by the glycan chains attached to Asn74 and Asn111 (both are glycosylated in insect cells [21] ); however, this EpEX form is cleaved almost to the same extent as the non-glycosylated EpEXΔ ( Supplementary Fig. 5 ). This suggests that proteases act on monomeric EpEXΔ or on a loosened cis -dimer where the cleavage site within the TY loop would be more accessible. Translated to the cell surface EpCAM, this would mean that there is a dynamic equilibrium between monomeric and dimeric EpCAM as already indicated [11] . Another possibility is that the TM helix dimer stays intact and that the extracellular parts temporarily move apart to a certain degree giving protease opportunity to access the identified cleavage site. The monomer–dimer equilibrium could be affected by various factors, such as lipid composition or association with other proteins. Also, the EpEX dimer could be destabilized by a pH drop, which we already demonstrated in vitro [28] . A locally acidic environment with pH even below 6.5 (ref. 41 ) is often found in tumours and could at the same time maintain the activity of various proteolytic enzymes released into the extracellular space. Even more, while EpCAM is not expected to be a physiological substrate of trypsin and other proteases used in previous studies, the lysosomal cysteine cathepsins used in our study are under some conditions released to the extracellular space where they actively participate in ECM remodelling or even ECM degradation, for example in cancer (reviewed in ref. 42 ). Therefore, it is tempting to speculate that they are involved in in vivo EpCAM cleavage affecting the oligomeric state, associated functions and turnover of EpCAM at the cell surface. The slight differences in observed cleavage site (Gly79-Arg80 as observed with cathepsins L and K, and Arg80-Arg81 as reported previously [33] ) could be a result of further N-terminal trimming at Gly79 or action of different proteases at this protease-sensitive region in different cells. In humans, EpCAM is heterogeneously glycosylated at the three N -glycosylation sites [43] and it has been demonstrated that glycosylation at Asn198 is crucial for stability [30] . As inferred from the model of glycosylated EpEX ( Fig. 2c ), this glycosylation site is located close to the membrane where it might influence trafficking or interactions with proteins affecting EpCAM turnover rate. The arrangement of glycan chains attached to Asn111 and Asn198 in the cis -dimer resembles the tripod-like arrangement of glycans in the membrane-proximal region of ICAM-2 where they are assumed to play a role in a proper orientation of ICAM-2 with regard to the cell surface and interacting cells [44] . This is also in line with our model of the intercellular EpCAM trans -tetramer ( Fig. 5 ). This model suggests sporadic intercellular contacts unlike the extensive contacts based on a zipper-like model of the C-cadherin junctions [45] . Comparison of the interaction surface between two subunits in the EpEXΔ cis -dimer (2,438 Å 2 ) and between two cis -dimers in our model of the trans -tetramer (800 Å 2 ) is also in line with the determined dissociation constants (~10 nM and ~10 μM for dimer-to-monomer and tetramer-to-dimer, respectively) [11] . The high dissociation constant for the tetramer-to-dimer equilibrium is in compliance with the absence of tetramer in crosslinking experiments ( Fig. 3a ). In cells, the tetramer-to-dimer equilibrium could be strongly affected by the crowding effect in the intercellular space along with the restricted degrees of freedom due to membrane anchoring. However, in case of conformational changes in the RCD a different relative orientation of the two dimeric subunits could be favored. Also, the conformation of RCD in our structure could be imposed by the bound n-decyl-β- D -maltopyranoside ( Supplementary Fig. 2 ). The amino-acid sequence of EpEX is highly conserved in organisms like primates, ungulates and rodents, and to a certain extent even in other groups of organisms such as fishes, amphibians and reptilians ( Supplementary Fig. 3a ). Specifically, the most conserved parts are the core of the TY (α1 helix and the region including the βB) and the secondary structure elements of the CD (except the α2 helix). Also, in organisms ranging from primates through ungulates and rodents to birds, reptiles and amphibians the TY-loop region is largely conserved including the dibasic site (Arg80-Arg81 in humans). Since the βC and the TY loop are critically involved in cis -dimerization, it is reasonable to assume that also in all these organisms EpEX also forms a cis -dimer. Interestingly, fishes have a four to six amino-acid residue insertion in this region indicating a somewhat different cis -dimerization mechanism if even applicable. Sequence conservation mapped to the structure of EpEX cis -dimer revealed that most differences lie in the membrane-distal part of the dimer ( Supplementary Fig. 3b ). This region, which is formed by the ND and the α2 helix plus RCD of the CD, may represent the environment-sensing part of EpCAM while the lateral parts may be involved in interactions with other (trans)membrane proteins on the surface of the same cell. In the light of this information, the RCD and possibly the nearby α2 are proposed to be directly involved in EpCAM trans -tetramerization as described in our paper. An important aspect of EpCAM biology is the proteolytic release of EpIC, which is implicated in proliferative signalling. Since the cleavage of cell surface EpCAM could be triggered by soluble EpEX added to the cell culture, it was suggested that formation of intercellular oligomeric units is a prerequisite or a trigger for the initial cleavage event [19] . The formation of a trans -tetramer could be accompanied by conformational changes, which are translated to the C-terminal region of the extracellular part close to the membrane resulting in cleavage-promoting structural changes. To date, several cleavage sites were identified. For example, it has been reported that in bladder cancer patients, EpEX is shed via cleavage at the Ala266-Gly267 site [46] corresponding to the beginning of the EpCAM TM part. This cleavage would directly release the EpEX from the cell surface since it would break the membrane anchoring provided by the TM region. In mouse, other cleavage sites were observed, which in human EpCAM correspond to Ser228-Lys229 (α-site, close to the βD within the RCD, Fig. 1b ), Tyr250-Tyr251 (β-site, within the βC4, Fig. 3b ), and several sites within the TM region including the γ 2 - and γ 1 -sites Ala270-Val271 and Val273-Val274, respectively ( Fig. 4c ) [47] . The α-cleavage site within the RCD would imply that the protease active site is at least 5 nm from the cell surface as inferred from the EpEX dimensions or is a result of proteolytic action of a protease at the surface of a neighbouring cell or even a soluble protease. While the α-site appears accessible in the cis -dimer, the β-cleavage within βC suggests a dynamic equilibrium between EpCAM monomer and cis -dimer (discussed above) since in the cis -dimer this cleavage site is inaccessible. It is tempting to speculate that the β-cleavage is triggered by a local drop of pH since this both destabilizes the EpEX cis -dimer and at the same time enhances the activity of the BACE1 protease involved in the cleavage [47] , [48] . However, both cleavages within the CD as identified using murine EpCAM seem to be incompatible with the model where the formation of trans -intercellular contacts triggers the signalling-associated cleavage. The intramembrane cleavages, particularly at both γ-sites, could interfere with TM helix dimerization since this region is located at the crossing region of the TM helix dimer as predicted by MD simulations ( Fig. 4c ). However, the γ-cleavages are preceded by the cleavages within the extracellular part therefore we speculate that the cleavage-induced destabilization of the extracellular region conformationally and/or sterically paves the way for γ-cleavages within the TM part. Recently, additional cleavage sites at the extracellular part were identified: a cleavage at the mouth of the central groove in cis -dimer within a region connecting the βC1 to the α2 helix of the CD, and a several cleavages within and near the SCD ( Figs 1b and 2a ) [49] . The role of all these cleavages and the exact mechanism by which they occur remains to be elucidated. The structure of EpEXΔ also addresses the effect of CTE-causing mutations on EpCAM structural integrity. Most of the CTE-associated mutations within the EpCAM gene result in truncated forms of EpCAM lacking most of the CD along with TM and EpIC (reviewed in ref. 7 ), and only two result in an EpCAM molecule impaired in some other way—lacking either the Trp143-Thr164 region (corresponding to α2 helix and one of the two middle strands in βC sheet; Fig. 1b ) or having the Cys66 within TY mutated to Tyr [50] . The deletion most probably significantly impairs EpCAM folding by linking together two residues, which are more than 20 Å apart in the wt EpCAM. The second mutation results in the absence of a stabilizing disulphide bond between Cys66 and Cys99 ( Fig. 3b ) and also introduces a residue with a bulkier side chain seriously perturbing the core of the TY. This latter mutation could impair formation of EpCAM cis -dimers or even prevent normal folding of EpCAM and adoption of the compact overall structure. Another disease-associated aspect is the use of EpCAM as prognostic tool and for targeted drug delivery. The exceptional antigenicity of the ND has been recognized some time ago [34] and is in line with the location of this domain at a very exposed position in the EpEXΔ cis -dimer ( Figs 2a,c and 6 ). Moreover, the majority of epitopes mapped to this domain are destroyed by reduction of disulphide bonds confirming their conformational nature dependent on correct pattern of disulphide bonds within the compact ND. Other known polypeptide epitopes are primarily located in the membrane-distal or upper lateral part of the EpEXΔ cis -dimer, which is again in line with their higher accessibility due to lack of glycan chains and greater cell membrane–epitope distance ( Fig. 6 ). In addition, the membrane-proximal surface regions could be masked by other (interacting) membrane proteins. Still, while the ND is targeted by a plethora of antibodies, some surface-exposed regions of the TY and CD domain remain unexplored. Also, dissociation of the EpCAM dimer as speculated above would reveal additional potential epitopes previously located within buried surface and therefore inaccessible. Interestingly, the epitope of the HO-3 antibody, which is the EpCAM-binding part of the EU-approved Catumaxomab [6] extends from the part of ND through TY loop to part of the CD. This suggests that the HO-3 antibody/Catumaxomab recognizes EpCAM in a cis -dimeric form. At the same time, the epitope size indicates that antibody regions adjacent to the complementarity determining regions are involved in EpCAM recognition. In our model, the epitope of HO-3 is partially covered with glycan chains, which are, however, flexible and could move from the mentioned areas thereby exposing the polypeptide epitope ( Fig. 6 ). 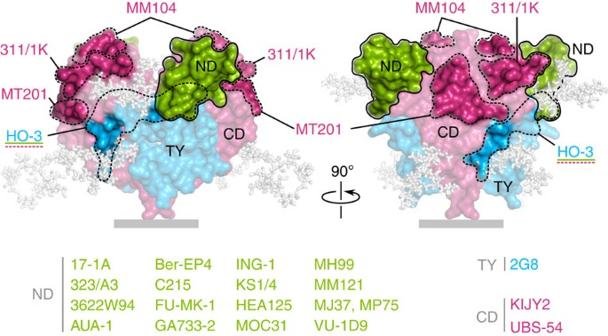Figure 6: Epitopes of anti-EpEX antibodies mapped to a pale-coloured surface model of glycosylated EpEXcis-dimer. The identified epitope regions and the most antigenic N-domain are depicted as intensively shaded surface regions. Listed below are other anti-EpEX antibodies for which the exact epitope is unknown. Antibody names are color-coded by the domains they recognize (ND, TY and CD in green, blue and dark pink, respectively). Epitopes of antibodies HO-3, 17-1A and MT201 are targeted by Catumaxomab, Edrecolomab and Adecatumumab, respectively. Figure 6: Epitopes of anti-EpEX antibodies mapped to a pale-coloured surface model of glycosylated EpEX cis -dimer. The identified epitope regions and the most antigenic N-domain are depicted as intensively shaded surface regions. Listed below are other anti-EpEX antibodies for which the exact epitope is unknown. Antibody names are color-coded by the domains they recognize (ND, TY and CD in green, blue and dark pink, respectively). Epitopes of antibodies HO-3, 17-1A and MT201 are targeted by Catumaxomab, Edrecolomab and Adecatumumab, respectively. Full size image In recent years, the EpCAM paralogue Trop2, the only other member of the GA733 family, is gaining attention as a stem [51] and carcinoma cell marker [52] . The two proteins share a 49% sequence identity and for Trop2 a signalling function via regulated intramembrane proteolysis reminiscent of EpCAM was demonstrated [53] . However, no adhesive function has been reported to date. It is important that the similarities/differences are taken into account when developing diagnostic/prognostic and therapeutic approaches and great care is needed when analysing the results with regard to both EpCAM and Trop2. Expression, purification and crystallization We prepared two EpEX variants— wt EpEX (residues 24-265 of EpCAM) and the non-glycosylated mutant variant (EpEXΔ), both with an uncleavable His 6 -tag at the C terminus. Briefly, the region of EpCAM cDNA (clone ID IRAKp961G0321Q; Source BioScience imaGenes) coding for Gln24-Lys265 was amplified by PCR. In case of EpEXΔ three mutations were introduced: Asn74Gln, Asn111Gln and Asn198Gln. Next, 5′- and 3′-ends of the DNA fragment were extended by PCR to introduce the N-terminal melittin signal peptide (MKFLVNVALVFMVVYISYIYA) and a C-terminal His 6 -tag. The resulting fragment was cloned into pFastBac1, which was in turn used to prepare recombinant baculoviruses using the Bac-to-Bac system (Invitrogen). Expression was performed using suspension cultures of Spodoptera frugiperda Sf9 cells at multiplicity of infection of 5. The recombinant protein was collected from the medium 36 h post infection by dialysis and subsequent immobilized metal affinity chromatography using Ni 2+ -charged HisTrap columns (GE Healthcare). The peak eluate fractions were pooled and EDTA (pH 8.0) was added to a final concentration of 5 mM. Following dialysis and ion-exchange chromatography on Mono Q column (GE Healthcare), the final buffer exchange was done by size-exclusion chromatography on a Superdex 200 column (GE Healthcare) equilibrated in 20 mM Na-HEPES pH 8.0, 100 mM NaCl. The peak fraction was pooled and concentrated using Amicon centrifugal filter unit with 10 kDa cutoff membrane (Millipore). EpEX was prepared using the same procedure; however, the ion-exchange chromatography step was omitted. This recombinant EpEX variant is heterogeneously glycosylated as revealed by the presence of multiple bands on SDS–polyacrylamide gel electrophoresis (SDS–PAGE) gel, all at higher M r than the EpEXΔ variant ( Supplementary Fig. 1a ). For crystallization only EpEXΔ was used due to higher sample homogeneity ( Supplementary Fig. 1a ). EpEXΔ was crystallized by sitting drop vapour diffusion at 295 K. Here, 2 μl of protein solution (10 mg ml −1 ) was mixed with 2 μl of crystallization buffer and 0.4 μl of 18 mM n-decyl-β- D -maltopyranoside. The crystallization buffer consisted of 0.1 M Tris–HCl (pH 8.5), 0.2 M magnesium chloride and 30% w/v PEG 4000. Crystals appeared within 25 days and reached dimensions 0.2 mm × 0.3 mm × 0.4 mm ( Supplementary Fig. 1b ). X-ray data collection and processing EpEXΔ crystals were directly flash-frozen in a stream of cool nitrogen (100 K). Screening and data collection were performed on an in-house Bruker AXS Microstar rotating copper anode X-ray generator (wavelength of 1.542 Å) equipped with Platinum 135 CCD detector. Images were processed using the PROTEUM2 Software Suite (Bruker AXS Inc.). The statistics for crystallographic data collection are presented in Table 1 . Structure determination and refinement The structure of EpEXΔ was determined by single-wavelength anomalous dispersion by intrinsic sulphur atoms (S-SAD) using highly redundant data set collected from a single crystal. The same data set was used in refinement. Initial data analysis was done in XTRIAGE [54] and showed the presence of one polypeptide chain per asymmetric unit. Positions of anomalous scatterers and initial phases were determined by HySS [55] . Here, the positions of 14 of the total 16 intrinsic sulphur atoms were resolved (12 sulphur atoms of the 6 disulphide bridges and 2 sulphur atoms of Met69 and Met73) while the sulphur atoms of surface-exposed Met231 and Met261 could not be resolved due to side chain disorder ( Supplementary Fig. 1c ). The initial model was built using AutoBuild [56] implemented in PHENIX [54] . The complete model was built with Arp/wArp [57] , [58] , [59] . The N-terminal residue (Gln in expressed construct) was modelled as pyroGlu based on the shape of electron density blob and previous reports [21] . The N-terminal Gln residue observed previously indicates that small amount of expressed protein has an unmodified N-terminal Gln residue resulting in QEExVxE N-terminal amino-acid sequence of purified EpEXΔ [28] . A large extended blob in the positive difference electron density map was identified as a crystallization additive n-decyl-β- D -maltopyranoside based on the shape of the blob and composition of the crystallization drop. The final model was produced after rounds of manual building in COOT [60] and refinement in PHENIX [54] . The quality of the final model was assessed by using MolProbity [61] . The Ramachandran plot distribution analysis revealed that 95.4% of residues are in the favored region and 4.6% in allowed region with no outliers. Refinement statistics are summarized in Table 1 . Structure analysis Protein structures with similar folds were identified using the protein structure comparison service PDBeFold at the European Bioinformatics Institute [23] . The model of glycosylated EpEX was prepared using GlyProt [62] . In this model, high-mannose chains were attached to the three asparagine residues known to be involved in otherwise heterogeneous wt glycosylation [30] to get a visual insight into the glycosylated molecule. Secondary structure assignments used in structure figures were performed using STRIDE [63] . All structure figures were prepared in PyMOL (Schroedinger) except those in Fig. 4b and Supplementary Fig. 3b that were prepared in VMD [64] . Amino-acid sequence alignment was prepared using ClustalW [65] . Sequence identity as inferred from the amino-acid sequence alignment was mapped to EpEXΔ structure using the MultiSeq 2.0 plugin [66] . MD simulation The EpCAM TM part with amino-acid sequence A 266 GVIAVIVVVVIAVVAGIVVLVI 288 was modelled as a canonical α-helix with acetyl N-terminal and N-methylamide C-terminal caps. Two such helices were embedded in 1-palmitoyl-2-oleoylphosphatidylcholine lipid bilayer patch of dimensions 100 Å × 100 Å. Helical axes were oriented perpendicularly to bilayer plain and the interhelical distance was set to 50 Å. This all-atom system was parameterized to a CG system using MARTINI force field and solvated [67] . Here, small groups of atoms (for example, amino-acid side chains) are treated as single particles allowing calculation of longer time scales. CG MD simulations were performed in NAMD 2.9 (ref. 68 ) using periodic boundary conditions and 10 fs time step under constant temperature (310 K) and pressure (1.01325 bar) controlled using Langevin dynamics. First, the protein part of the system was fixed and the lipids were allowed to equilibrate for 1.25 ns with stepwise harmonic restraints scaling. Next, the equilibrated system was used as a starting point for six independent 2-μs simulations using the same parameters. Obtained trajectories were analysed and visualized in VMD [64] and Gromacs [69] . The interhelical distance was defined as the distance between centres of the two helices. The interhelical crossing angle was defined as the angle between vectors describing the two helices; vector of each helix was drawn between centres of two groups of backbone atoms (Ala270-Val273 and Ala281-Val284). To right-handed orientation, a negative value vas assigned. Proteolytic cleavage EpEX and EpEXΔ were incubated with human recombinant cathepsins L, S, K and B. For each enzyme, a HEPES buffer with pH 7.2 and an additional low-pH buffer were used (sodium acetate pH 5.5 or Bis-Tris pH 6.0). All buffers were 0.1 M and contained 2 mM EDTA and 2 mM DTT. Cathepsin/EpEX(Δ) molar ratio was 10 −2 or 10 −3 . Reaction mixtures were incubated at 37 °C for 1 h. Reactions were stopped by adding reducing SDS–PAGE sample buffer followed by boiling. Fragments were visualized on 15% SDS–PAGE by Coomassie staining. Cleavage site was determined by N-terminal amino-acid sequencing (Edman degradation) of electrophoretically separated fragments transferred to a polyvinylidene difluoride membrane. Chemical crosslinking Crosslinking of intact or trypsin-cleaved EpEXΔ was performed in PBS by treating the protein with 1.3 mM BS 3 (Pierce) at 21 °C for 30 min. BS 3 has a spacer length of 11.4 Å. The reaction was quenched by adding Tris buffer (pH 7.4) to a final concentration of 50 mM followed by 30 min incubation at 21 °C. Reaction mixtures were analysed on 15% SDS–PAGE under non-reducing and reducing conditions. Protein bands were visualized by Coomassie staining. Docking Two EpEXΔ cis -dimers (chain labels A and B in one dimer and C and D in second dimer) were used in docking experiments to construct a model of the trans -tetrameric unit. Calculations were performed using HADDOCK running on WeNMR grid [70] . The N-terminal pyroGlu residue was changed to Gln because modified residues are not generally accepted in docking simulations. Histidine protonation states and flexible segments were defined automatically and centre of mass restraint was used to enforce contact between the molecules. C2 point symmetry restraint was imposed between the two dimers (AB–CD). An additional calculation was performed where C2 point symmetry restrains between subunits in each subunit pair (A–C, A–D, B–C, B–D) were used to limit calculation results to tetrameric units with perpendicular C2 rotation axes. Docking solutions were first ranked according to their HADDOCK and Z -scores, the latter indicating separation of a cluster of solutions from the average in terms of score (better solutions have more negative Z -scores), and further ranked according to the buried surface area and contacts between ND. Both docking runs yielded similar results. In the models from the best docking cluster ( Z =−1.2), the relative angle between the two cis -dimers was 30°, while in the models from second ( Z =−0.9) and third best clusters ( Z =0.1), the relative angle was 150° (ND’s already in contact) and 75°, respectively, with a smaller buried surface area. For figure preparation, the best model from additional symmetry-restrained docking run was used. Accession codes : Coordinates and structural factors have been deposited in the Protein Data Bank under accession code 4MZV . How to cite this article : Pavšič, M. et al. Crystal structure and its bearing towards an understanding of key biological functions of EpCAM. Nat. Commun . 5:4764 doi: 10.1038/5764 (2014).